An acetylome peptide microarray reveals specificities and deacetylation substrates for all human sirtuin isoforms Sirtuin enzymes regulate metabolism and aging processes through deacetylation of acetyl-lysines in target proteins. More than 6,800 mammalian acetylation sites are known, but few targets have been assigned to most sirtuin isoforms, hampering our understanding of sirtuin function. Here we describe a peptide microarray system displaying 6,802 human acetylation sites for the parallel characterisation of their modification by deacetylases. Deacetylation data for all seven human sirtuins obtained with this system reveal isoform-specific substrate preferences and deacetylation substrate candidates for all sirtuin isoforms, including Sirt4. We confirm malate dehydrogenase protein as a Sirt3 substrate and show that peroxiredoxin 1 and high-mobility group B1 protein are deacetylated by Sirt5 and Sirt1, respectively, at the identified sites, rendering them likely new in vivo substrates. Our microarray platform enables parallel studies on physiological acetylation sites and the deacetylation data presented provide an exciting resource for the identification of novel substrates for all human sirtuins. Reversible lysine acetylation is a post-translational protein modification rivalling phosphorylation in its ubiquitous occurrence and function [1] . More than 6,800 acetylation sites are known in the mammalian proteome, affecting a wide range of proteins, from histones to metabolic enzymes [2] . Protein acetylation is regulated by protein acetyl transferases and protein deacetylases. Sirtuins form deacetylase class III, which differs from other classes in the consumption of one nicotinamide adenine dinucleotide (NAD + ) cosubstrate per deacetylation [3] , coupling sirtuin activity to cellular energy levels. Sirtuins regulate central physiological functions, such as metabolism and cell cycle, and have been implicated in aging processes [4] . They are thus considered attractive targets for the treatment of metabolic and aging-related diseases [5] . Our knowledge on the seven mammalian sirtuin isoforms, Sirt1–7, differs widely, in particular with respect to in vivo substrates and functions [6] . The best studied isoform Sirt1, as well as isoforms 6 and 7, are located in the nucleus. More than 20 Sirt1 substrates are known, such as histones and transcription factors [6] . Sirt6 regulates DNA stability and repair [7] , and histone H3 and ‘C-terminal-binding protein-interacting protein’ were identified as first deacetylation substrates [8] , [9] . Sirt7 regulates RNA polymerase I [10] and can deacetylate p53 and histone H3 [11] , [12] . Sirt3, 4 and 5 are located in mitochondria [13] . Sirt3 influences stress responses and deacetylates many metabolic enzymes, whereas carbamoylphosphate synthetase 1 (CPS1) constitutes the only confirmed physiological Sirt5 deacetylation substrate [14] , [15] , [16] . Recently, Sirt5 was found to display stronger desuccinylase and demalonylase activity and to desuccinylate CPS1 at a Lys that can carry both succinylations and acetylations [17] . For Sirt4, no deacetylation substrate has yet been identified. Instead, Sirt4 was reported to regulate glutamate dehydrogenase through ADP-ribosylation [18] , an alternative, normally less efficiently catalysed reaction of sirtuins [19] . The major cytosolic isoform is Sirt2, which deacetylates, for example, α-tubulin [20] . The differently localized sirtuins contribute to a spatially varying regulation of protein acetylation, and the key for deciphering sirtuin function is identification of their target proteins. Crystal structures of several sirtuins have revealed their conserved catalytic core architecture [21] . NAD + and acetyl-Lys enter the active site from a cleft between a Rossmann fold domain and a smaller, structurally more variable Zn 2+ -binding domain. The peptide binding grooves are architecturally conserved but exhibit isoform-specific features such as charge distribution and shape details. Although certain sirtuins appear to lack sequence specificity, most studies find sirtuin selectivity for substrates with certain residue types around the deacetylation site [22] , [23] , [24] . Such studies were restricted however to a limited number of sirtuins and few substrate peptide sequences. A characterisation of all human sirtuins against a large set of physiological acetylation sites, revealing specificities and potential in vivo substrates, is lacking. Here we describe a peptide microarray system enabling parallel characterisation of deacetylation activities against several thousand human acetylation sites. Testing all human sirtuins reveals isoform-specific sequence preferences and novel in vitro substrates, including first deacetylation substrates for Sirt4. Exemplarily, we confirm deacetylation of a Sirt3 substrate candidate and of target sites identified in the novel Sirt1 and Sirt5 substrates high-mobility group B1 (HMG-B1) and peroxiredoxin 1 (Prx1), respectively, with complete proteins as substrates. These results demonstrate that the microarray data reveal excellent candidates for physiological sirtuin substrate proteins. Acetylome-wide deacetylation assays using microarrays For hypothesis-free assignment of substrates from the many known mammalian acetylation sites to the seven human sirtuins, we established a peptide microarray system for parallel studies on human acetylation sites. Collecting published acetylation sites in human proteins and at conserved sites in proteins from other mammals resulted in 6,802 sites ( Supplementary Data 1 and 2 ). 13meric peptides comprising six residues N- and C-terminal from the acetylation sites were synthesized in acetylated and non-acetylated form. Peptide length was based on previous results indicating that four residues up- and downstream of the acetyl-Lys dominate sirtuin/substrate recognition [23] , [24] . Acetylome microarrays were generated by immobilization of these peptides via the N terminus onto modified glass slides. For quality control, all 13,604 peptides were spotted in triplicates ( Fig. 1a ) resulting in 40,812 features displayed on two microarrays. 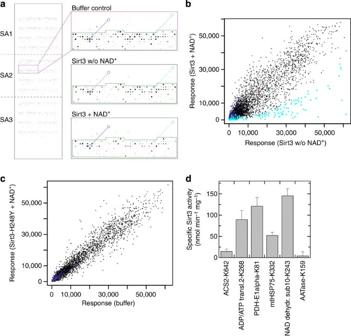Figure 1: Deacetylation assay for the acetylome microarray established with human Sirt3. (a) Fluorescence image of three identical subarrays (SA1–SA3) of an acetylome microarray treated with Sirt3 buffer control (left), and comparison of the same sector of subarray 2 (magenta frame) from chips either treated with buffer control (top right) or Sirt3 in the absence (middle) or presence (bottom) of NAD+. Sections with acetylated peptides are framed in green. Examples for non-acetylated and acetylated variants of substrate candidates are marked in blue and cyan. (b) Scatter plot of signals after Sirt3 treatment with (yaxis) or without (xaxis) NAD+. Sirt3 substrates show a significant signal decrease versus control (cyan circles) shifting them to the lower right. Signals of non-acetylated control peptides are plotted as blue squares. (c) Scatter plot for treatment with inactive Sirt3-His248Tyr versus Sirt3 buffer control. For details see panel b. (d) Sirt3 deacetylation assays in solution with peptides harbouring potential Sirt3 substrate sites. The known Sirt3 substrate ACS2-Lys642 and AAT-Lys159 (not deacetylated on array) are included for comparison. Representative of two repetitions; error bars: s.d. of linear fits to time series with four data points. Figure 1: Deacetylation assay for the acetylome microarray established with human Sirt3. ( a ) Fluorescence image of three identical subarrays (SA1–SA3) of an acetylome microarray treated with Sirt3 buffer control (left), and comparison of the same sector of subarray 2 (magenta frame) from chips either treated with buffer control (top right) or Sirt3 in the absence (middle) or presence (bottom) of NAD + . Sections with acetylated peptides are framed in green. Examples for non-acetylated and acetylated variants of substrate candidates are marked in blue and cyan. ( b ) Scatter plot of signals after Sirt3 treatment with ( y axis) or without ( x axis) NAD + . Sirt3 substrates show a significant signal decrease versus control (cyan circles) shifting them to the lower right. Signals of non-acetylated control peptides are plotted as blue squares. ( c ) Scatter plot for treatment with inactive Sirt3-His248Tyr versus Sirt3 buffer control. For details see panel b. ( d ) Sirt3 deacetylation assays in solution with peptides harbouring potential Sirt3 substrate sites. The known Sirt3 substrate ACS2-Lys642 and AAT-Lys159 (not deacetylated on array) are included for comparison. Representative of two repetitions; error bars: s.d. of linear fits to time series with four data points. Full size image First, we used the acetylome microarray to test generic anti-acetyl-Lys antibodies, which should be sequence-insensitive but in fact show varying preferences for flanking residues [25] . We found a large variation of signal intensities for different peptides ( Fig. 1a–c ; Supplementary Data 3 ), and that different subsets of peptides were recognized by each antibody ( Supplementary Data 4 ). The acetylome microarray thus is an excellent tool for pan anti-acetyl-Lys antibody characterisation. Our results also show that an optimized mix of three antibodies ( Supplementary Data 4 and 5 ) enables recognition of almost all microarray peptides, and it was thus used in deacetylation experiments. Fluorescence signals were generated by adding two labelled secondary antibodies. Generally, weak fluorescence signals were obtained for non-acetylated peptides and stronger signals for acetylated peptides ( Fig. 1a ). Signals for acetylated peptides showed good correlation between different microarrays ( Supplementary Fig. S1 ), and only for 220 of the 6,802 peptide pairs no significant signal difference could be obtained ( Supplementary Data 6 ). For deacetylation assays, microarrays were treated with the sirtuin of interest before adding antibodies. As a first test, we treated an acetylome microarray either with recombinant human Sirt3 in presence of NAD + or with a buffer control ( Fig. 1a ). Sirt3 treatment decreased a specific set of signals compared with buffer control, and correlation coefficients for signals from identical peptides in three different subarrays were usually >95% ( Supplementary Data 5 ; Supplementary Fig. S2 ). To ensure that signal changes were due to the NAD + -dependent deacetylation activity of Sirt3 rather than a contaminating enzyme from the expression host or other artifacts we performed additional controls. Sirt3 treatment in the absence of NAD + resulted in largely unchanged signals, confirming that the deacetylation is NAD + -dependent ( Fig. 1a,b ). Furthermore, we tested a catalytically inactive Sirt3 variant (Sirt3-H248Y) expressed and purified identical to the active Sirt3. No significant signal changes were observed when Sirt3-H248Y was compared with a control without protein solution added (buffer control; Fig. 1c ), confirming that signal changes are caused by recombinant Sirt3 and not by a contaminating E. coli deacetylase. Additionally, we stained a Sirt3-treated microarray with anti-Sirt3-antibody and fluorescently labelled secondary antibody. No signals were detected, confirming that signal decreases in the anti-acetyl-Lys antibody experiments are caused by deacetylation and not through masking of the epitope by bound sirtuins, consistent with results of a previous test for sirtuin binding to a peptide array [24] . We conclude that the peptide microarray system is suitable for the highly parallel analysis of deacetylation of known acetylation sites by purified mammalian sirtuins for specificity studies and substrate candidate identification. Human Sirt1-7 have different substrate preferences Our deacetylation assay is based on a loss of signal, which makes small changes hard to measure. Therefore, we refrained from a detailed interpretation of signal ratios treated/reference ( Supplementary Data 1 ; errors represent variations between peptide spot triplicates and experiment repetitions), which were calculated for comparison of deacetylations since reference signals varied between peptides (see above). For finding potential deacetylation substrates, we identified peptides with significant signal loss using Welch’s t -test ( Supplementary Data 3 ) and combined these results from experiment repetitions in a ‘substrate category’ value ( Supplementary Data 1 ), which represents a deacetylation likelihood between 0 and 1. To ensure that peptidic Sirt3 substrates found on the microarray are substrates in homogeneous assays, we tested peptides in solution using mass spectrometry. 13meric peptides representing (de)acetylation sites in mitochondrial heat shock protein 75 (mtHsp75; Lys332), pyruvate dehydrogenase (PDH) subunit E1α (Lys81), NADH dehydrogenase 1α subunit 10 (Lys243) and ADP/ATP translocase 2 (Lys268) were efficiently deacetylated by Sirt3 ( Fig. 1d ). Deacetylation efficiencies in solution showed good, albeit not quantitative correlation to relative deacetylation levels on the array ( Supplementary Fig. S3 ). An aspartate aminotransferase (AATase; Lys159) peptide showed no significant deacetylation in solution, consistent with its lack of deacetylation by Sirt3 on the microarray ( Fig. 1d ). Thus, deacetylation of microarray-displayed peptides enables identification of peptidic substrates in solution, yielding insights into sequence preferences and candidates for physiological deacetylation targets. We next used the microarrays to determine preferred substrates for all seven human sirtuins. Recombinant Sirt1 through 7 ( Supplementary Fig. S4 ; Supplementary Data 5 ) were tested on microarrays, and controls without NAD + (and additionally of an inactive mutant for Sirt1) confirmed again that signal changes were caused by the respective deacetylase activity ( Supplementary Data 1 and 5 ). For Sirt1, 6 and 7, constructs of catalytic core with or without outside domains showed no significant differences ( Supplementary Fig. S5 ), consistent with the embedment of the substrate binding cleft in the catalytic core, and results were thus aggregated to maximize coverage of sequence space deacetylated by the respective isoform. Comparing the panels of peptides deacetylated by each sirtuin isoform based on their efficiency (category/ratio, Supplementary Data 1 ) showed only partial overlap ( Fig. 2a ). This comparison cannot show which isoform will dominantly deacetylate a site, as different enzyme amounts had to be used due to different intrinsic activities (see Discussion), but it reveals differences in substrate sequence preferences. Nuclear Sirt6 and Sirt7, for example, show overlapping preference for a small set of peptides but unique activity against most of their substrates, and even less overlap is observed for the mitochondrial isoforms Sirt3 and Sirt5 ( Fig. 2a ). Inherent substrate preferences of human sirtuins thus allow selection of specific substrates. However, differences are observed between Sirt1-7 in the distribution of strong and weak deacetylation. Sirt2, for example, shows strong activity against a broad, but still defined, range of sites, whereas Sirt1 shows a more even activity distribution. Sirt2 thus shows stronger sequence selectivity than Sirt1. We conclude that each human sirtuin has its unique sequence preference and that their sets of deacetylation substrate sites show only partial overlap. Thus, sirtuins can at best partially compensate for other isoforms in knockout experiments. 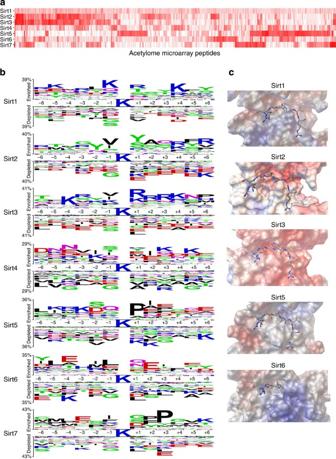Figure 2: Substrate sequence preferences of human sirtuins and molecular features of their substrate-binding sites. (a) Map of deacetylation efficiencies (red, high efficiency; white, low efficiency) for all seven human sirtuins (vertical axis) and the 6,802 peptides on the microarray (horizontal axis). (b) Two Sample Logos for the 50 peptides with highest deacetylation efficiency for each sirtuin, with all other peptides used as negative set. Favoured residues are above, disfavoured residues below the bars (center: acetyl-Lys; see scalable PDF of this paper for the small letters). (c) Comparison of peptide binding grooves of human sirtuins. Surfaces were calculated from crystal structures (Sirt2, -3, -5 and -6) or a homology model (Sirt1). Peptide binding grooves are indicated by the peptide of an experimentally determined Sirt3/peptide complex, which was transferred to the other sirtuins through overlays. Colour indicates the electrostatic potential (red: negative; blue: positive). Figure 2: Substrate sequence preferences of human sirtuins and molecular features of their substrate-binding sites. ( a ) Map of deacetylation efficiencies (red, high efficiency; white, low efficiency) for all seven human sirtuins (vertical axis) and the 6,802 peptides on the microarray (horizontal axis). ( b ) Two Sample Logos for the 50 peptides with highest deacetylation efficiency for each sirtuin, with all other peptides used as negative set. Favoured residues are above, disfavoured residues below the bars (center: acetyl-Lys; see scalable PDF of this paper for the small letters). ( c ) Comparison of peptide binding grooves of human sirtuins. Surfaces were calculated from crystal structures (Sirt2, -3, -5 and -6) or a homology model (Sirt1). Peptide binding grooves are indicated by the peptide of an experimentally determined Sirt3/peptide complex, which was transferred to the other sirtuins through overlays. Colour indicates the electrostatic potential (red: negative; blue: positive). Full size image Substrate sequence subsite preferences of human sirtuins To characterise in detail the substrate preferences of the human sirtuins, we analysed statistically the sequences of the deacetylation substrates identified on the microarray ( Fig. 2b ). The preferences of nuclear isoforms Sirt1 and Sirt6 differ strongly, showing that sirtuins with the same subcellular localization still select specific targets. Sirt1 prefers polar, mainly positively charged residues surrounding the deacetylation site ( Fig. 2b ), with non-charged residues inserted at positions +2, +3 and −2. These features correlate with the hydrophilic Sirt1 peptide binding groove, negatively charged on the bottom, as indicated by a Sirt1 homology model ( Fig. 2c ). Sirt6, in contrast, prefers non-charged residues, with the exception of negatively charged residues at +2 and −4 ( Fig. 2b ). The general preference for less polar residues, in particular hydrophobic ones at −1/−2 and +3/+4, and disfavouring of positive charges in many positions are consistent with the largely hydrophobic peptide binding site with a positive patch on the front ( Fig. 2c ). Consistently, we observed weak Sirt6-dependent deacetylation of the hydrophilic histone H3-Lys56 peptide, in agreement with the described weak deacetylation of this site [8] , [26] . Our results indicate that better physiological deacetylation substrates for Sirt6 should exist and provides candidate sites for testing (see below). The third nuclear isoform, Sirt7, shows a preference for hydrophilic non-charged or negatively charged residues, especially in positions −3, −2 and +1 ( Fig. 2b ). In positions +2 to +5 and −4/−5, less hydrophilic residues are favoured, and positions +2/+3/−2 show a preference for Pro. We also find distinct sequence preferences for the mitochondrial isoforms Sirt3, 4 and 5. Sirt3 prefers positively charged and disfavours negatively charged residues downstream of the deacetylation site and—less pronounced—in several upstream positions, consistent with the negative electrostatic potential of the Sirt3 peptide binding cleft ( Fig. 2c ). The profile compares well to a Sirt3 binding preference from iterative refinement of an array of 300 peptides [24] . Differences in detail, such as a higher preference for large hydrophobic residues from the approach of Smith et al . [24] , might have technical reasons, such as testing binding versus turnover (our assay). For Sirt5, we find a strong preference for Pro in +1 and a weaker preference for negatively charged downstream residues, and hydrophilic non-charged or positively charged residues upstream, except for −2 ( Fig. 2b ). As the stronger Sirt5 activity desuccinylation affected a Lys found with both modifications, acetylation and succinylation [17] , we speculate that succinylation and acetylation sites overlap and that the Sirt5 sequence preference applies to both acylations. Consistent with our Sirt5 sequence preference, Sirt5 structures show that the peptide binding cleft is a partly hydrophobic groove with positively charged patches in the pocket for downstream residues ( Fig. 2c ). Sirt4, in contrast, favours hydrophobic residues in −2 and shows weak preference for negatively (−4/+1/+2/+4) or positively (+3/+5) charged residues in the other, hydrophilic positions. Sirt4 is thus unique among mitochondrial isoforms in having a more subtle deacetylation sequence preference than Sirt5 and Sirt3, which mainly favour positively (Sirt3) or negatively (Sirt5) charged substrates. The cytosolic Sirt2 disfavours negatively charged residues ( Fig. 2b ), especially downstream, consistent with its polar peptide binding cleft with largely negatively charged bottom, especially on the downstream side ( Fig. 2c ). A slight disfavouring of negatively charged residues is also observed for Sirt1, which is mainly nuclear but was also found in the cytosol [27] . However, Sirt2 favours positively charged residues only at +4 and slightly on the N terminal side, resulting in cytosolic Sirt2 activity clearly distinct from potential cytosolic Sirt1. Potential sirtuin substrate proteins and target pathways Analysis of the microarray hits revealed several known sirtuin/substrate pairs, such as p300-Lys418 for Sirt2 and histones for Sirt1. Three of the four known Sirt1 histone deacetylation sites [28] were deacetylated (H3-Lys9, H3-Lys14 and H1-Lys26), only H4-Lys16 was not recognized. Microarray hits thus can indicate target proteins ( Fig. 3a ; Supplementary Data 1 and 7 ), enabling focused follow-up studies for verification of physiological sirtuin substrates. For Sirt1, significant deacetylation was also observed for novel candidate sites in known substrates, for example, Lys21 of histone H4, and in novel substrate protein candidates, such as transcription factor IID subunit 3 (TFIID; Lys625) and HMG-B1 (Lys12; Supplementary Data 1 ). Testing these peptides in solution resulted in deacetylation efficiencies similar (HMG-B1-Lys12) or higher (TFIID3-Lys625) than against the known substrate site p53-Lys382 ( Fig. 3b ). No significant deacetylation was observed for AATase-Lys159 as a negative control (no significant deacetylation on the microarray). Thus, HMG-B1-Lys12 and TFIID3-Lys625, if accessible within the full-length proteins (see below), should serve as Sirt1 substrate sites. 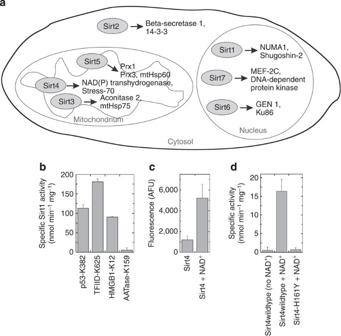Figure 3: Novel substrates for human sirtuins indicate target sites. (a) Cellular localization of the seven mammalian sirtuins and newly identified substrate candidates residing in the same compartment (Sirt5 was detected in both, mitochondrial matrix and intermembrane space). (b) Sirt1-dependent deacetylation tested in solution using a continuous coupled enzymatic assay. Peptides representing novel substrate candidates HMG-B1-Lys12 and TFIID-Lys625 were deacetylated with similar efficiency as the peptide representing the known substrate p53-Lys382 (AATase-Lys159: negative control). Representative of three replications; error bars: s.d. of linear fits to time courses with 250 data points. (c) Sirt4 deacetylates the fluorogenic Fluor-de-Lys 1 substrate peptide in an NAD+-dependent manner. Representative of two replications; error bars: s.d. of triplicates. (d) Sirt4 deacetylates a peptide representing the substrate site candidate Nnt-Lys397 in presence, but not in the absence of NAD+. The catalytically inactive mutant Sirt4-H161Y has no effect on the acetylation level. Representative of two repetitions; error bars: s.d. of linear fits to time series with five data points. Figure 3: Novel substrates for human sirtuins indicate target sites. ( a ) Cellular localization of the seven mammalian sirtuins and newly identified substrate candidates residing in the same compartment (Sirt5 was detected in both, mitochondrial matrix and intermembrane space). ( b ) Sirt1-dependent deacetylation tested in solution using a continuous coupled enzymatic assay. Peptides representing novel substrate candidates HMG-B1-Lys12 and TFIID-Lys625 were deacetylated with similar efficiency as the peptide representing the known substrate p53-Lys382 (AATase-Lys159: negative control). Representative of three replications; error bars: s.d. of linear fits to time courses with 250 data points. ( c ) Sirt4 deacetylates the fluorogenic Fluor-de-Lys 1 substrate peptide in an NAD + -dependent manner. Representative of two replications; error bars: s.d. of triplicates. ( d ) Sirt4 deacetylates a peptide representing the substrate site candidate Nnt-Lys397 in presence, but not in the absence of NAD + . The catalytically inactive mutant Sirt4-H161Y has no effect on the acetylation level. Representative of two repetitions; error bars: s.d. of linear fits to time series with five data points. Full size image To identify candidates for novel target proteins and pathways of Sirt1 through 7, we thus sorted their hit lists according to the deacetylation likelihood or ratio, respectively. Several peptides could be excluded as representing physiological substrates due to different cellular localizations of sirtuin and target, but we refrained from correcting the hit lists ( Supplementary Data 1 ), as protein localization annotations are sometimes unreliable, and because sirtuin isoform localization seems to be complex [29] , [30] . Yet, we also listed for each sirtuin the top 12 hits from proteins known to exist in the same compartment ( Supplementary Data 7 ) and focused the following description of substrate and target pathway candidates ( Fig. 3a ) on such proteins because we consider them the most likely in vivo substrates. For Sirt1, proteins involved in transcription regulation are among the top hits, such as Mediator subunit 1 (Lys1504). Furthermore, proteins contributing to chromosome structure and condensation, such as Nuclear mitotic apparatus protein 1 (NUMA1; Lys2071) and Shugoshin-2 (Lys385) indicate a Sirt1 function in chromosome segregation. For Sirt6, novel potential targets contributing to its function in stress responses and DNA repair [7] , [9] include the endonuclease GEN1 (Lys230), and Ku subunits p86 (Lys665, -195 and -155) and p70 (Lys468). Ku70 is a known Sirt1 substrate, indicating that target regulation by different sirtuins might integrate signalling pathways. Further hits, such as phosphatidylinositol-4-phosphate 5-kinase (Lys145), indicate Sirt6 connections to other signalling pathways. For Sirt7, we identified in p53, its only known substrate protein besides histone H3 [11] , [12] , Lys382 as a strongly deacetylated site (also a Sirt1 substrate site [6] ). Novel potential substrates include transcription factors (for example, Myocyte-specific enhancer factor 2C, MEF-2C; Lys239) and DNA-dependent protein kinase (Lys117), indicating that Sirt7 regulates DNA structure and function. Putative Sirt7 substrates such as A-kinase anchor protein 8 (Lys538) and hnRNP-R (Lys369) indicate additional functions, for example, in cAMP signalling and RNA processing. For mitochondrial Sirt3, a known metabolic regulator, we find additional metabolic enzymes as potential substrates ( Fig. 3a ; Supplementary Data 1 and 7 ), such as aconitase 2 (Lys50) and mitochondrial malate dehydrogenase (MDH; Lys239,335). Further identified targets likely contribute to the Sirt3 function in stress response [29] , [31] , such as the mitochondrial heat shock proteins mtHsp60 (Lys473, -469 and -156) and mtHsp75 (Lys332). For Sirt5, the best mitochondrial substrates are from the metabolic enzymes medium-chain acyl-CoA dehydrogenase (Lys212, 279, 301) and hydroxymethylglutaryl-CoA synthase 2 (Lys437), and from heat shock proteins mtHsp70 (Lys234) and mtHsp60 (Lys462, -130, -82 and 125). These hits indicate that Sirt5 can influence lipid metabolism and stress responses. Interestingly, the mtHsp60 sites are complementary to those deacetylated by Sirt3. Furthermore, hydroxymethylglutaryl-CoA synthase 2 is a known Sirt3 target [32] , again indicating that sirtuin targets could serve as signalling integration points (see above) and/or that different sirtuins might remove different acylations, such as acetylation and succinylation, which appear to affect the same target residues [17] . A Sirt5 function in stress response would be consistent with the hits Prx3 (Lys83, 93) and Prx1 (Lys197). Prx1 resides in the mitochondrial intermembrane space (besides a cytosolic fraction) [33] , which contains reversibly acetylated proteins [34] and no deacetylase other than Sirt5 [13] , [16] . For Sirt4, no deacetylation substrate has been reported yet. Instead, Sirt4 can ADP-ribosylate histones and GDH [18] , but this activity might have been observed as only activity due to the lack of proper deacetylation substrates. Indeed, we detected low but reproducible Sirt4 deacetylation activity against the non-physiological Fluor-de-Lys peptide ( Fig. 3c ). Consistently, Sirt4 showed significant deacetylation activity on our acetylome microarray revealing candidates for physiological deacetylation substrates. Top hits are mtHsp60 (Lys31) and Stress-70 (Lys135, 595), which has been implicated in cell proliferation and aging, as well as NAD(P) transhydrogenase (a.k.a. nicotinamide nucleotide transhydrogenase, Nnt; Lys394, 331, 397), an enzyme important for redox stress responses. Testing Nnt-Lys397 peptide in solution confirmed its deacetylation by Sirt4 in a NAD + -dependent manner, while no deacetylation was observed for the catalytically inactive variant Sirt4-His161Tyr ( Fig. 3d ). The hits indicate that Sirt4 may contribute to stress responses and constitute excellent candidates for identifying in vivo deacetylation targets. For cytosolic Sirt2, our microarray identified substrate candidates possibly mediating Sirt2 contributions to neuronal function and diseases [35] , [36] , such as beta-secretase 1 (Lys126). Additional candidates include ubiquitin-conjugating systems (E3 protein RING2 Lys249; Ubiquitin carboxyl-terminal hydrolase 14 Lys313) and 14-3-3 adapter proteins (for example, 14-3-3 β/α Lys117), indicating functions in regulating protein homoeostasis and signal transduction. Protein deacetylation substrates for human sirtuins Our microarray displays peptides derived from in vivo acetylation sites, and deacetylation by a sirtuin thus indicates candidates for physiological substrates. Several hits are known sirtuin substrates, confirming that our approach allows finding in vivo substrates. We thus tested identified substrate and substrate site candidates for their deacetylation in context of the full-length target protein. First, we tested deacetylation of the Sirt3 substrate candidate mitochondrial MDH, isolated from native source, by using an ELISA. Sirt3 reduced MDH acetylation levels, and the effect was impeded by adding the sirtuin inhibitor nicotinamide ( Fig. 4a ). These results cannot identify the acetylation site affected, but they confirm that Sirt3 can deacetylate native MDH protein. Sirt3-dependent MDH deacetylation in vivo was indeed confirmed during the revision of this manuscript [37] . The site identified in this proteomics study, Lys239, corresponds to the MDH microarray peptide most efficiently deacetylated by Sirt3, demonstrating the suitability of our system for identifying promising sirtuin substrates and substrate sites. 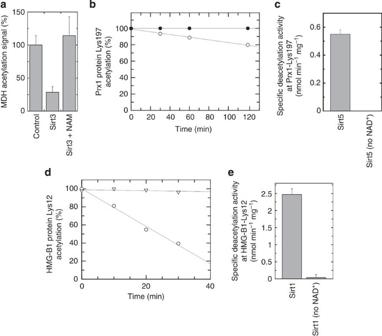Figure 4: Experimental analyses of substrate candidates for human sirtuins. (a) ELISA experiment showing that Sirt3 deacetylates full-length MDH protein, an effect suppressed by the sirtuin inhibitor nicotinamide (NAM). Representative of three replications; error bars: s.d. of triplicates. (b) Time-course for deacetylation of Prx1 protein, specifically acetylated at Lys197, by human Sirt5 (). A control without cosubstrate () confirmed the NAD+dependence. Representative of two replications. (c) Reaction rates obtained from the time-courses in (b). Error bars: s.d. of linear fits to time series with four data points. (d) Time-course for Sirt1-dependent deacetylation of HMG-B1-Lys12 in the presence () and absence of NAD+(). Representative of two replications. (e) Reaction rates obtained from the time-courses in (d). Error bars: s.d. of linear fits to time series with four data points. Figure 4: Experimental analyses of substrate candidates for human sirtuins. ( a ) ELISA experiment showing that Sirt3 deacetylates full-length MDH protein, an effect suppressed by the sirtuin inhibitor nicotinamide (NAM). Representative of three replications; error bars: s.d. of triplicates. ( b ) Time-course for deacetylation of Prx1 protein, specifically acetylated at Lys197, by human Sirt5 ( ). A control without cosubstrate ( ) confirmed the NAD + dependence. Representative of two replications. ( c ) Reaction rates obtained from the time-courses in ( b ). Error bars: s.d. of linear fits to time series with four data points. ( d ) Time-course for Sirt1-dependent deacetylation of HMG-B1-Lys12 in the presence ( ) and absence of NAD + ( ). Representative of two replications. ( e ) Reaction rates obtained from the time-courses in ( d ). Error bars: s.d. of linear fits to time series with four data points. Full size image We next analysed CPS1, the only confirmed physiological Sirt5 deacetylation substrate, whose acetylation sites responsible for Sirt5-dependent activation have not been identified [15] . The array experiments identified among eight CPS1 acetylation sites (Lys55, -119, -287, -527, -841, -869, -892 and -1291) Lys119 and Lys527 as the best Sirt5 substrates ( Supplementary Data 1 ). A CPS1-Lys527 peptide can indeed be deacetylated in solution [38] , and a homology model for human CPS1 N-terminal domain ( Supplementary Fig. S6 ) based on an E. coli CPS1 crystal structure [39] indicates an accessible surface position for CPS1-Lys119, suggesting these sites as regulatory switches responsible for Sirt5-dependent activation of human CPS1. To analyse a new Sirt5 substrate predicted from our array experiments, we then tested Sirt5-dependent deacetylation of full-length Prx1. Prx1 protein specifically acetylated at Lys197, the site most sensitive to Sirt5 on microarrays, was prepared by native chemical ligation ( Supplementary Fig. S7 ) and its deacetylation tested using mass spectrometry. Sirt5 catalysed the time-dependent deacetylation of Prx1 protein at Lys197, and no deacetylation was observed in a control without NAD + ( Fig. 4b,c ). This result provides an example for identification of a sirtuin substrate site in a native protein based on our microarray data. Deacetylation of Prx1-Lys197, also catalysed in the cytosol by HDAC6, induces the low peroxidase activity form of Prx1 [40] , [41] . It will be exciting to see whether this target, like CPS1 (ref. 17 ), can also be (de)succinylated at this site, and whether Sirt5 contributes to redox signalling and stress responses through deacylation of the mitochondrial intermembrane space fraction of Prx1 (ref. 33 ). We next tested deacetylation of the Sirt1 substrate candidate HMG-B1. Sirt1 catalysed the NAD + -dependent deacetylation of recombinant, acetylated HMG-B1 protein at Lys12 ( Fig. 4d,e ), which had been identified as a top Sirt1 substrate site in peptide microarray experiments ( Supplementary Data 7 ). These results provide an additional example for a sirtuin substrate and substrate site identified from our peptide microarray data and confirmed as a substrate on the protein level. In conclusion, microarray experiments enable the efficient identification of sirtuin substrate sites in native proteins. Microarray hits thus represent excellent candidates for physiological deacetylase targets, and our hit lists for human Sirt1-7 will serve as a valuable resource for the identification of in vivo sirtuin substrates. Protein acetylation sites are often dynamically modified in response, for example, to nutrients [34] , [42] . The metabolically regulated sirtuins should catalyse many of these deacetylations—for example, in mitochondria, where no other deacetylase families have been found—but few substrates have been assigned to most sirtuins [6] , leaving the mechanisms unclear how they influence physiological processes. Our acetylome microarrays enabled the characterisation of sirtuin substrate specificities and provide excellent candidates for sirtuin substrates, enabling a hypothesis-free approach for the identification of novel in vivo substrates and target pathways. Even acetylation sites not yet reported and thus not displayed on the microarray can be proposed as targets based on the identified sequence preferences. Another peptide array approach to Sirt3 characterisation used iterative synthesis/testing of a smaller number of peptides and machine-learning for guiding subsequent synthesis cycles [24] . It yielded improved Sirt3 substrates and some sequences resembled physiological acetylation sites. Our approach requires synthesis of a larger peptide collection but does not rely on any—possibly inaccurate—models and yields a direct read-out for all sequences, which all represent physiological acetylation sites. The model-based approach, in contrast, might be advantageous for understanding specificity contributions of individual substrate residues. However, the Sirt3 substrate profiles from both approaches are very similar, indicating that our Sirt1-7 specificities not only depict preferences among known acetylation sites but also their general sequence preferences, as expected due to the large variation of sequences analysed in our study. Our microarray assays yielded different numbers of strongly deacetylated peptides for different isoforms. This discrepancy could be caused by different enzymatic activities—due to different intrinsic activities and reflected by the different enzyme amounts used—or by more restricted specificities of some isoforms. Isoform activities cannot be compared easily as each of the substrates has individual K M and k cat values for each sirtuin, preventing data normalization to a common reference. However, the substrate category values allow preference comparisons between isoforms, and their variation among microarray peptides indicates how strictly substrates are defined. Analyses of our results indicate that both different activities and differently strict specificities have a role. Sirt3, for example, appears to have higher average activity than Sirt4, and Sirt1 seems to be less specific than most other isoforms indicated by a more even distribution of deacetylation efficiencies ( Fig. 2a ). However, basal sirtuin activity is likely regulated in vivo by ligands and post-translational modifications, such as their known phosphorylations [43] , and it will be exciting to study such effects using our microarrays. A further contribution to observed differences could stem from sequence bias of the anti-acetyl-Lys antibodies [25] . They could preferentially recognize a subset of peptides more suitable for a certain sirtuin. However, identification of many substrate peptides and different specificities for each isoform show that the microarray covers sufficient sequence space for meaningful results on sequence preferences of all isoforms. Sirtuin crystal structures and peptide tests (Cosgrove et al . [23] , Smith et al . [24] and references therein) indicate that substrate recognition is dominated by four to five target residues N- and C-terminal from the acetyl-Lys, which bind through backbone interactions and surface contacts rather than side-chain insertions in defined sirtuin pockets. Consistently, we find a moderate sequence preference and a strong influence of substrate polarity in specific positions. More distant residues, not covered by our peptides, might also influence deacetylation through interactions with the sirtuin or by influencing the conformation of the acetyl-Lys region, and false positives could result from limited accessibility of a good substrate site in the full-length protein. Each deacetylation site thus has to be confirmed on native target protein and ultimately in vivo . However, microarray sites were selected based on their acetylation in vivo , which shows that they are accessible for acetylation, and thus likely also for deacetylation, within the target protein. In fact, several hits corresponded to previously confirmed substrate sites, and our tests on selected novel target proteins exemplarily confirm the accessibility of newly identified sites in native proteins. We conclude that our microarrays are powerful tools for specificity studies and hypothesis-free identification of substrate candidates for sirtuins and other protein deacetylases, enabling new insights in targets and processes regulated by reversible acetylation. Chemicals and peptides Chemicals were from Sigma (Saint Louis, Missouri, USA) if not stated otherwise. HPLC-purified peptides for assays were from GL Biochem (Shanghai, China). Preparation of human Sirt1-7 protein Human Sirt1 residues 1–747 and 225–664, Sirt2-34-356, Sirt3-114-399 and 114-380, Sirt4-25-314, Sirt5-34-302, Sirt6-13-308 and 13–355, and Sirt7-1-400, 59–356, and 14–367 were expressed with N-terminal His-tag in E. coli [29] , [44] , [45] . Proteins were purified through affinity and size exclusion chromatography (see also Supplementary Methods ). Inactive variants Sirt3-His248Tyr, Sirt1-His363Ala, and Sirt4-His161Tyr were generated by site-directed mutagenesis and purified as the respective wild-type protein. Manufacturing of human acetylome peptide microarrays Peptides were synthesized in parallel on cellulose membranes using SPOT technology [46] , [47] . After each coupling, remaining amino functions were acetylated using acetic anhydride in DMF in presence of DIPEA to prevent deletion sequences. A linker (N-(3-(2-(2-(3-amino-propoxy)-ethoxy)-ethoxy)-propyl)-succinamic acid) was added to the peptides as Fmoc-protected derivative followed by an acetylation step. After Fmoc removel with 20% piperidine in DMF, coupling with anthranilic acid-transformed full-length peptides with free N terminus, but not N-terminally acetylated, truncated side products from incomplete coupling, into 2-aminobenzoyl-derivatives. Following side chain deprotection, peptides were transferred into 96-well filtration plates (Millipore, Bedford, Massachusetts, USA) and cleaved from cellulose through treatment with 200 μl 2.5% ( v / v ) triethylamine. Peptide solution was filtered off and quality controlled by LC-MS. Solvent was evaporated under reduced pressure, and peptide derivatives (50 nmol) were dissolved in 25 μl printing solution (70% DMSO, 25% 0.2 M sodium acetate, 5% glycerol, pH 4.5; by volume) and transferred into 384-well microtiterplates. Microarrays were generated by contact printing on epoxy-modified slides (PolyAn; Berlin, Germany). Our buffer conditions resulted in selective covalent bond formation between epoxy-functions and amino groups of 2-amino-benzoyl-derivatives; control experiments with fluorophore-labelled peptides without aminobenzoyl-function but containing other potentially reactive groups (amino, thiol, or hydroxyl functions) showed dramatically reduced binding (fluorescence decrease >90%). Microarrays were quenched and washed with water followed by ethanol, resulting in ‘purified peptide’ spots, essentially free of deletion sequences (due to acetylation steps during synthesis) and truncated sequences (due to chemoselective immobilization). Printed microarrays were dried using a microarray centrifuge and stored at 4 °C. To ensure similar loadings between spots, a >100-fold excess of peptide derivative (5 pmole) over reactive groups on the glass (150 fmol mm −2 ) was used, which provides sufficient peptide derivative for maximal loading even for sequences with low yield during synthesis. Microarray-based deacetylation assays Peptide microarrays were treated for 2 h in the presence or absence of 6–218 μg ml −1 sirtuin in reaction buffer ( Supplementary Data 5 ), washed with water and dried in a chip centrifuge. The following steps were performed in a HS400 hybridization station (Tecan, Männedorf, Switzerland) at 25 °C, with washing steps of 2 min purging and 2 min soaking. Microarrays were washed 3 × with TBST (20 mM Tris, 150 mM NaCl, 0,1% Tween20, pH 8.0) and once with TBS (20 mM Tris, 150 mM NaCl, pH 7.5). They were incubated for 1 h with a mix of three primary antibodies ( Supplementary Data 5 ), washed with TBST (5 × ) and TBS (1 × ), and incubated 30 min with fluorophore-labelled secondary antibodies ( Supplementary Data 5 ). Microarrays were washed with TBST (5 × ) and water (2 × ), dried with nitrogen gas, and scanned at 10 nm resolution using a Genepix Scanner 4000B (Molecular Devices, Sunnyvale, USA) with a 635-nm laser. Spot recognition was done using Genepix Pro 7.0 (Molecular Devices) and a GAL-file from JPT Peptide Technologies (Berlin, Germany) and corrected manually with uncertain spots marked as ‘bad’. Array data processing was done in GNU R [48] . Spot signal was defined as the mean of foreground pixels. Correlation of subarrays was estimated for each chip ( Supplementary Data 5 ). Significance of fluorescence signals was tested using Welch’s t -test on unweighted means for acetylated and non-acetylated peptides, respectively. Peptides with P >0.05 and higher signals for the non-acetylated variant were marked as non-detectable ( Supplementary Data 4 ). Subarrays were normalized independently using an invariant method from R package ‘affy’ [49] , [50] with proportion rank differences of 0.003 and 0.008 and a buffer-only microarray as reference. Subarrays were aggregated as means weighted with reciprocals of the in-spot-variance ( Supplementary Data 3 ). For determination of sirtuin substrates, P -values of Welch’s t -test and signal ratios for peptides of a sirtuin-treated microarray and those of a reference microarray treated with inactive mutant, active sirtuin without NAD + or buffer-only were used. Peptides with significant loss of signal ( P <0.01) were categorized as potential substrates and combined as substrate category in Supplementary Data 1 . Ratios from multiple experiments for the same sirtuin were summarized using weighted means. The ratio of the count of substrates to ‘anti-substrates’ (gain of signal) was used as weight to favour experiments with low scattering and many substrate candidates. Quotients of category and ratio (efficiency) were used for cluster analysis and heat map preparation using fastcluster (D. Müllner, fastcluster: Fast hierarchical clustering routines for R and Python ; http://math.stanford.edu/~muellner ). For each sirtuin the 50 peptides with highest efficiency values (marked in Supplementary Data 1 ) were used as positive set to prepare Two Sample Logos [51] , with all other peptides as negative set. No significance was set to show all amino acids. Deacetylation assays Continuous coupled deacetylation assays [52] were done with 0.64 mM substrate peptide, 1 mM NAD + and 1 μM Sirt1. Fluor-de-Lys assays were done according to the manufacturer’s protocol (Enzo Life Sciences, Farmingdale, New York, USA) with 100 μM Fluor-de-Lys-2 peptide, 1 mM NAD + and 7 μg Sirt4. For ELISA-based deacetylation tests [29] , 200 μg MDH purified from mitochondria (Sigma) were used for coating and 0.5 mM NAD + and 5 μg Sirt3 for deacetylation. Mass spectrometry peptide deacetylation assays in 10 μl 20 mM Tris/HCl pH 7.8, 150 mM NaCl, 0.5 (Sirt3) or 1 mM NAD + (Sirt4) and sirtuin protein (Sirt3: 1 μg; Sirt4: 20 μg) were started with 0.5 mM substrate peptide, incubated at 37 °C, and stopped after certain times (Sirt3: 5/10/15/30 min; Sirt4: 0/15/30/60/120 min) with trifluoroacetic acid (0.25% ( v / v )). Samples were diluted with 0.1% ( v / v ) formic acid to 1 pmol μl −1 peptide, filtered and measured by LC-ESI-MS (see below). Deacetylation of specifically acetylated Prx1or chemically acetylated HMG-B1 was assayed by the incubation of 94 μM Prx1 or 97 μM HMG-B1 with 9.4 μM Sirt5 (Prx1) or 9.7 μM Sirt1 (HMG-B1) and 2.5 mM NAD + in 20 mM Tris/HCl, 150 mM NaCl (pH 7.8) at 37 °C. Reactions were stopped after 0/30/60/120 min (Prx1) or 0/10/20/30 min (HMG-B1) with 5 mM nicotinamide, and the protein digested with trypsin (trypsin to protein ratio 1: 20) in 25 mM NH 4 HCO 3 (pH 8.5), 5 mM nicotinamide for 4 h at 37 °C. Peptides were reduced (10 mM DTT, 30 min at 37 °C) and alkylated (20 mM iodoacetamide, 20 min in the dark at RT) and the digest stopped with trifluoroacetic acid (final concentration 5% ( v / v )). Samples were filtered and measured by LC-ESI-MS using single reaction monitoring (SRM). For LC-ESI-MS analyses on a prominence HPLC (Shimadzu, Duisburg, Germany) connected to a LTQ-XL mass spectrometer (Thermo Fisher, Bremen, Germany), 2 pmol peptide or 9 pmol digested Prx1 or HMG-B1 protein was injected in a trapping column (Phalanx C18 5 μm, Higgins analytical) and separated on a homemade 100-μm ID capillary reversed phase column (Dr Maisch, Reprosil C18 AQ, 3 μm) using a linear gradient from 0 to 45% buffer B (buffer A: 0.1% TFA, 0.02% HFBA; buffer B: 70% ACN, 0.1% TFA, 0.02% HFBA) [38] . Full MS scans, followed either by MS/MS scans of the three most intensive ions or by three SRMs (to monitor Prx1-Lys197 and HMG-B1-Lys12) were acquired. Transitions were selected using Skyline Software [53] . The heated desolvation capillary was set to 180 °C and dynamic exclusion was enabled with a repeat count of 1 and a 1 min exclusion duration window. Peptide quantification was done in Xcalibur 2.1. Extracted ion chromatograms were generated for acetylated and deacetylated peptides with mass windows of ±2 m / z [38] , or the respective scan filters were applied in case of SRM measurements, and the Xcalibur automatic peak area detection was then used. Acetyl-HMG-B1 and specifically acetylated Prx1 preparation HMG-B1 amino acids 1–84 were expressed in E. coli and acetylated with acetic anhydride (see Supplementary Methods ). Prx1 residues 1–195 were expressed in E. coli as intein-fusion with an N-terminal His-tag. Affinity-purified Prx1-intein fusion was cleaved with 300 mM sodium 2-mercaptoethanesulfonate [54] , and the obtained protein-thioester was ligated with synthetic C-terminal Prx1 peptides CKQK and C(acetylK)QK, respectively. For details see Supplementary Methods . Homology modelling and analysis of sirtuin structures A homology model for human Sirt1 residues 214–497 (UniProt entry Q96EB6) was generated with Modeller [55] based on an alignment with human Sirt2-34-356 (PDB entry 3ZGO [56] ). Crystal structures of Sirt2 [56] , Sirt5 (PDB ID 2B4Y) [57] and Sirt6 (3K35) [58] and the Sirt1 homology model were superimposed on the structure of a Sirt3/peptide complex (3GLR) [59] , and electrostatic potentials were calculated with Adaptive Poisson–Boltzmann Solver and mapped on the surface in python molecule viewer [60] . How to cite this article: Rauh, D. et al . An acetylome peptide microarray reveals specificities and deacetylation substrates for all human sirtuin isoforms. Nat. Commun. 4:2327 doi: 10.1038/ncomms3327 (2013).